Human copper chaperone for superoxide dismutase 1 mediates its own oxidation-dependent import into mitochondria Oxidative stress is counteracted by various cellular systems, including copper–zinc superoxide dismutase 1 (SOD1) and its activating chaperone, that is, the copper chaperone for SOD1 (CCS1). Both enzymes are structurally related, and both localize to the cytosol and the mitochondrial intermembrane space where they specifically counteract mitochondria-derived superoxide. The mechanism by which human CCS1 is transported into mitochondria is largely unclear. Here we show that CCS1 import depends on the presence of mature CCS1 in the mitochondria. During import, a disulphide bond is formed in CCS1 in a CCS1-dependent reaction. We demonstrate that oxidation and import depend on the presence of cysteine residues at positions 227 and 141/144 in CCS1. Notably, CCS1 import parallels SOD1 import that also depends on CCS1. Our observations suggest that CCS1 serves as a specialized import receptor in mitochondria that facilitates the import and folding of SOD1 and CCS1, thereby extending the substrate spectrum of oxidation-dependent protein import in the mitochondrial intermembrane space. In eukaryotic cells, reactive oxygen species (ROS) mainly originate from the single electron reduction of molecular oxygen (O 2 ) at the respiratory chain [1] . The resulting superoxide anion (O 2 − ) is highly reactive and might damage molecules like iron–sulphur clusters. In vivo , it is rapidly dismutated into O 2 and hydrogen peroxide (H 2 O 2 ) by superoxide dimutases (SODs) [1] . H 2 O 2 has a longer half-life than O 2 − , which enables it to react with a variety of molecules causing, for example, cysteine oxidation, but also producing more deleterious hydroxyl radicals [2] , [3] . H 2 O 2 is removed by enzymes, such as peroxiredoxins, glutathione peroxidase and catalases. Importantly, ROS act not only as damaging agents but are also known to be important signalling molecules [4] , [5] . Thus, enzymes that react with ROS can also be considered as signal mediators and modulators. Mammals have three SODs with different subcellular localizations: SOD1 localizes to the cytosol and the intermembrane space of mitochondria (IMS); SOD2 localizes to the mitochondrial matrix; and SOD3 localizes to the extracellular matrix [6] . The subcellular localization of SOD activity may not only be important for the removal of O 2 − but could also contribute to the site-specific generation of the signalling molecule H 2 O 2 . As O 2 − is mainly generated by the respiratory chain, the localization of SOD1 to the mitochondrial IMS is especially interesting, because SOD1 might mediate a signalling pathway that communicates activity states of the respiratory chain and oxidative stress to the cytosol [7] , [8] . SOD1 requires an activating factor, the copper chaperone for SOD1 (CCS1), which introduces copper ions and disulphide bonds into SOD1 (ref. 9 ). Knockouts of CCS1 in Saccharomyces cerevisiae and in mouse result in hypersensitivity to oxidative stress due to the loss of SOD1 activity [10] , [11] , [12] . Similar to SOD1, CCS1 is present both in the cytosol and the IMS [13] . In S. cerevisiae , the specific elimination of CCS1 either from the cytosol or the IMS results in a loss of SOD1 activity in the respective compartments [14] , [15] , [16] , suggesting that localization of CCS1 controls the localization of SOD1 activity. Furthermore, several reports have shown that the translocation of SOD1 to the IMS depends on IMS-localized CCS1 (refs 13 , 14 ). Recently, we and others elucidated the mechanism of IMS import of S. cerevisiae CCS1 (scCCS1) [15] , [16] , [17] . scCCS1 is imported via the mitochondrial disulphide relay system [18] . Thereby, it traverses the outer mitochondrial membrane in an unfolded state and then interacts with the mitochondrial oxidoreductase Mia40, which forms a disulphide bond between two cysteine residues of scCCS1 (C27 and C64) [15] , [16] . This oxidative folding step traps scCCS1 in the IMS. The interaction between scCCS1 and Mia40 is relatively weak and, in vitro , the oxidation is slow compared with that of other substrates of Mia40. This likely explains why only a minor fraction of scCCS1 becomes imported into the IMS, while the majority folds in the cytosol. Dependence of CCS1 localization on Mia40 has also been reported in human cells [19] . However, human CCS1 (hsCCS1) does not contain cysteines that correspond to C27 and C64 in scCCS1. Thus, the mechanism of hsCCS1 import into the IMS remained unclear. In this study, we identify a novel oxidative import pathway into the mitochondrial IMS that is independent of Mia40. Import of hsCCS1 is hereby mediated by interactions with hsCCS1 molecules that are already present in the IMS. We also show that this process is accompanied by oxidation of cysteines in hsCCS1, which suggests that hsCCS1 distribution in the cell and, thus, SOD1 activity may be regulated by the redox conditions of the IMS. Different routes for CCS1 import into the human and yeast IMS Mitochondrial localization of scCCS1 depends on Mia40 (ref. 17 ) and the cysteine residues C27 and C64 of scCCS1 (refs 15 , 16 ; Fig. 1a ). However, these cysteines are not conserved and lack, for example, in animals, plants and many fungi, including Schizosaccharomyces pombe and Neurospora crassa ( Fig. 1b , Supplementary Fig. S1 ). hsCCS1 contains a serine and a threonine residue at the corresponding positions (S32 and T69; Supplementary Fig. S1 ). Still, studies on human and murine cells indicated that mammalian CCS1s also accumulate in the IMS [19] , [20] . To confirm these findings, we analysed the cellular distribution of hsCCS1 in HEK293 cells expressing carboxy-terminally haemagglutinin (HA)-tagged hsCCS1 (hsCCS1-HA), whose transcription is driven in a doxycycline-inducible manner ( Fig. 1c ). The majority of hsCCS1-HA was found in the cytosolic fraction, and a minor portion localized to the mitochondrial fraction. This confirms that cysteines corresponding to C27 and C64 of scCCS1 are not necessary for hsCCS1 to be imported into the IMS of HEK293 cells. 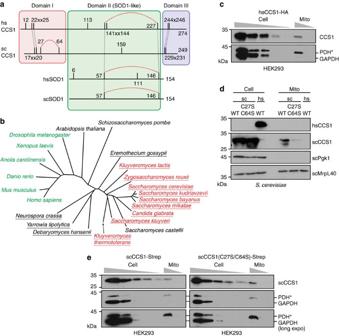Figure 1: CCS1 import pathways in human andS. cerevisiaerecognize different features of CCS1. (a) Schemes of human CCS1 (hsCCS1),S. cerevisiaeCCS1 (scCCS1), human SOD1 (hsSOD1) andS. cerevisiaeSOD1 (scSOD1). Positions of cysteine residues are indicated. Conserved cysteines are connected with grey dotted lines. Red dotted lines connect hypothetical or proven pairs of disulphide-forming cysteines. (b) Phylogenetic tree of CCS1. Species coloured in red contain cysteines corresponding to C27 and C64 of scCCS1. Green coloured species contain cysteines corresponding to C227 and C141 of hsCCS1. Underlined species contain proline residues at positions homologous to P144 of scSOD1 that determines the dependence of SOD1 activation on CCS1 (ref.9). For detailed information, seeSupplementary Fig. S1. (c) Cytosolic and mitochondrial fractions were prepared from hsCCS1-HA-expressing HEK293 cells by differential centrifugation and were loaded on SDS–PAGE in a five-time dilution series. Western blot analysis was performed using the indicated antibodies. Glyceraldehyde 3-phosphate dehydrogenase (GAPDH) and PDH served as cytosolic and mitochondrial loading controls, respectively. (d) scCCS1 (WT), scCCS1(C27S/C64S) and hsCCS1 were expressed inΔccs1strain ofS. cerevisiaeand mitochondria were isolated. Levels of CCS1 were analysed by western blotting. PGK1 and MrpL40 served as cytosolic and mitochondrial loading controls, respectively. (e) Total and mitochondrial protein extracts from HEK293 cells producing scCCS1 and scCCS1(C27S/C64S) were loaded on SDS–PAGE in a five-time dilution series. Protein levels were analysed by western blotting. Figure 1: CCS1 import pathways in human and S. cerevisiae recognize different features of CCS1. ( a ) Schemes of human CCS1 (hsCCS1), S. cerevisiae CCS1 (scCCS1), human SOD1 (hsSOD1) and S. cerevisiae SOD1 (scSOD1). Positions of cysteine residues are indicated. Conserved cysteines are connected with grey dotted lines. Red dotted lines connect hypothetical or proven pairs of disulphide-forming cysteines. ( b ) Phylogenetic tree of CCS1. Species coloured in red contain cysteines corresponding to C27 and C64 of scCCS1. Green coloured species contain cysteines corresponding to C227 and C141 of hsCCS1. Underlined species contain proline residues at positions homologous to P144 of scSOD1 that determines the dependence of SOD1 activation on CCS1 (ref. 9 ). For detailed information, see Supplementary Fig. S1 . ( c ) Cytosolic and mitochondrial fractions were prepared from hsCCS1-HA-expressing HEK293 cells by differential centrifugation and were loaded on SDS–PAGE in a five-time dilution series. Western blot analysis was performed using the indicated antibodies. Glyceraldehyde 3-phosphate dehydrogenase (GAPDH) and PDH served as cytosolic and mitochondrial loading controls, respectively. ( d ) scCCS1 (WT), scCCS1(C27S/C64S) and hsCCS1 were expressed in Δccs1 strain of S. cerevisiae and mitochondria were isolated. Levels of CCS1 were analysed by western blotting. PGK1 and MrpL40 served as cytosolic and mitochondrial loading controls, respectively. ( e ) Total and mitochondrial protein extracts from HEK293 cells producing scCCS1 and scCCS1(C27S/C64S) were loaded on SDS–PAGE in a five-time dilution series. Protein levels were analysed by western blotting. Full size image Does hsCCS1 contain motifs other than C27/C64 recognized by the import pathway? To answer this question, we compared the distributions of hsCCS1 and scCCS1 in human and S. cerevisiae cells. First, we analysed the localization of hsCCS1, scCCS1 and scCCS1(C27S/C64S) in S. cerevisiae ( Fig. 1d ). As expected, we detected a significant amount of wild-type (WT) scCCS1 but not of the C27S/C64S mutant in the mitochondrial fraction. Remarkably, hsCCS1 behaved similar to the C27S/C64S mutant and localized exclusively to the cytosolic fraction. The results suggest that the import pathway of CCS1 in S. cerevisiae requires some property of scCCS1 that is absent in hsCCS1—most likely C27 and C64. Next, we assessed the opposite situation—the subcellular distribution of scCCS1 in HEK293 cells. Independent of the presence of C27 and C64, a fraction of scCCS1 always localized to the mitochondria in HEK293 cells stably expressing the proteins ( Fig. 1e ). We estimated the ratio between cytosolic and mitochondrial scCCS1 to be around 100:1 to 100:5, which is comparable to that of hsCCS1-HA (compare Fig. 1c,e ). Taken together, our results indicate that the CCS1 import pathway in HEK293 cells recognizes different properties of CCS1 than the corresponding pathway in S. cerevisiae . Human CCS1 becomes oxidized in the mitochondrial IMS In scCCS1, C27 and C64 form a structural disulphide bond during IMS import. This disulphide bond is also formed—albeit much slower—in the S. cerevisiae cytosol [16] . As previous reports demonstrated a Mia40-dependence of hsCCS1 import, we wondered whether hsCCS1 also contains disulphide bonds in the IMS. To assess the redox state of hsCCS1 in the IMS, we constructed a HEK293 cell line expressing hsCCS1 fused to the amino-terminal 57 amino acid-long mitochondrial targeting signal (MTS) of human Smac/Diablo (Smac MTS -hsCCS1-HA) that drive the import of Smac into the IMS. Fusion with these 57 amino acids is sufficient to target non-IMS proteins to the IMS [21] , [22] . Indeed, we could confirm the mitochondrial localization of Smac MTS -hsCCS1-HA ( Fig. 2a ). Furthermore, cell fractionation based on digitonin treatment revealed that Smac MTS -hsCCS1-HA becomes released to the soluble fraction at digitonin concentrations that are lower than required to release the mitochondrial matrix protein, pyruvate dehydrogenase ( Fig. 2b ). Instead, Smac MTS -hsCCS1-HA became eluted like endogenous Smac verifying its IMS localization. 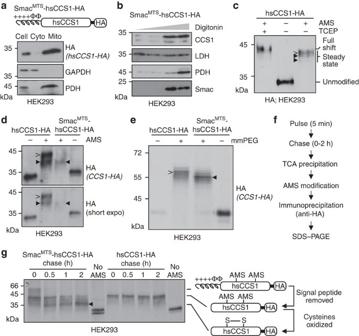Figure 2: Human CCS1 becomes oxidized in mitochondria. (a) Cytosolic and mitochondrial fractions were prepared from SmacMTS-CCS1-HA-producing HEK293 cells by differential centrifugation. Western blot analysis was performed using the indicated antibodies. Glyceraldehyde 3-phosphate dehydrogenase (GAPDH) and PDH served as cytosolic and mitochondrial loading controls, respectively. (b) HEK293 cells producing SmacMTS-CCS1-HA were treated with 0, 0.005, 0.03 and 0.3% (w/v) digitonin, and proteins released to the supernatant were analysed by SDS–PAGE and western blotting. Lactate dehydrogenase (LDH), PDH and Smac/Diablo served as loading controls for cytosol, mitochondrial matrix and IMS, respectively. (c) HEK293 cells producing hsCCS1-HA were treated with AMS to assess thein vivoredox state of hsCCS1. Changes in the molecular mass of hsCCS1 by alkylation were analysed by western blotting. Treatment with the reductant TCEP (tris-(2-carboxyethyl)phosphine) before alkylation leads to a modification of all cysteines in hsCCS1 and, consequently, to the maximally possible shift. Unmodified hsCCS1 represents a fully oxidized form of the protein in which no cysteines are accessible to AMS. (d,e) HEK293 cells producing hsCCS1-HA or SmacMTS-hsCCS1-HA were treated with AMS (d) or mmPEG24 (e). Changes in the molecular mass of hsCCS1 by alkylation were analysed by western blotting. (f) Outline of the experimental procedure for the ‘oxidation assay’. HEK293 cells producing hsCCS1-HA or SmacMTS-CCS1-HA were labelled with [35S] methionine for 5 min, followed by chase periods with cold methionine of 0 to 2 h. Cells were precipitated with TCA, and proteins were modified with AMS. HA-tagged proteins were isolated by IP assay and analysed by SDS–PAGE and autoradiography. As a control for unmodified (that is, oxidized CCS1), we left one sample that had been chased for 2 h unmodified. (g) Analysis of oxidative folding of hsCCS1-HA or SmacMTS-CCS1-HA. The experiment was performed as described inf. Original immunoblot images are shown inSupplementary Fig. S7. Figure 2: Human CCS1 becomes oxidized in mitochondria. ( a ) Cytosolic and mitochondrial fractions were prepared from Smac MTS -CCS1-HA-producing HEK293 cells by differential centrifugation. Western blot analysis was performed using the indicated antibodies. Glyceraldehyde 3-phosphate dehydrogenase (GAPDH) and PDH served as cytosolic and mitochondrial loading controls, respectively. ( b ) HEK293 cells producing Smac MTS -CCS1-HA were treated with 0, 0.005, 0.03 and 0.3% (w/v) digitonin, and proteins released to the supernatant were analysed by SDS–PAGE and western blotting. Lactate dehydrogenase (LDH), PDH and Smac/Diablo served as loading controls for cytosol, mitochondrial matrix and IMS, respectively. ( c ) HEK293 cells producing hsCCS1-HA were treated with AMS to assess the in vivo redox state of hsCCS1. Changes in the molecular mass of hsCCS1 by alkylation were analysed by western blotting. Treatment with the reductant TCEP (tris-(2-carboxyethyl)phosphine) before alkylation leads to a modification of all cysteines in hsCCS1 and, consequently, to the maximally possible shift. Unmodified hsCCS1 represents a fully oxidized form of the protein in which no cysteines are accessible to AMS. ( d , e ) HEK293 cells producing hsCCS1-HA or Smac MTS -hsCCS1-HA were treated with AMS ( d ) or mmPEG24 ( e ). Changes in the molecular mass of hsCCS1 by alkylation were analysed by western blotting. ( f ) Outline of the experimental procedure for the ‘oxidation assay’. HEK293 cells producing hsCCS1-HA or Smac MTS -CCS1-HA were labelled with [ 35 S] methionine for 5 min, followed by chase periods with cold methionine of 0 to 2 h. Cells were precipitated with TCA, and proteins were modified with AMS. HA-tagged proteins were isolated by IP assay and analysed by SDS–PAGE and autoradiography. As a control for unmodified (that is, oxidized CCS1), we left one sample that had been chased for 2 h unmodified. ( g ) Analysis of oxidative folding of hsCCS1-HA or Smac MTS -CCS1-HA. The experiment was performed as described in f . Original immunoblot images are shown in Supplementary Fig. S7 . Full size image Next, we assessed the redox states of hsCCS1-HA and Smac MTS -hsCCS1-HA by specifically modifying reduced cysteines with thiol-alkylating reagents that add weight to reduced but not oxidized cysteines. Consequently, a protein migrates slower on SDS–polyacrylamide gel electrophoresis (PAGE) in its reduced than in its oxidized form (compare, for example, lanes 1 and 2 in Fig. 2c ). First, we determined the redox state of hsCCS1-HA ( Fig. 2c ). As most hsCCS1-HA (95–99%) localizes to the cytosol ( Fig. 1c ), the detected redox state represents the redox state of hsCCS1-HA in the cytosol. After treatment with alkylating agents, hsCCS1-HA migrated as two to three bands on SDS–PAGE, all of which migrated slightly faster than fully modified (that is, reduced) hsCCS1-HA and much more slowly than unmodified hsCCS1-HA ( Fig. 2c ). This indicates that cytosolic hsCCS1-HA molecules contain at least one inaccessible cysteine, and that some hsCCS1-HA molecules might contain additional disulphide bonds. After alkylation, Smac MTS -hsCCS1-HA representing mitochondrial hsCCS1 migrated faster than hsCCS1-HA, indicating it to be more oxidized ( Fig. 2d,e , compare lanes 2 with 3). The data are similar to our previous findings for scCCS1 (ref. 16 ), which is more reduced in the cytosol than in the IMS. Similar to that for scCCS1, we propose that the cytosolic redox pools of hsCCS1 represent almost completely reduced hsCCS1 and hsCCS1 containing one or two disulphide bonds that form only slowly in the cytosol but rapidly in the IMS. To test whether mitochondrial hsCCS1 becomes oxidized faster than its cytosolic counterpart, we investigated the dynamics of the oxidation process. We thus followed the changes of the redox states of hsCCS1-HA and Smac MTS -hsCCS1-HA after synthesis by pulse-chase analysis in an oxidation assay ( Fig. 2f ). Using this assay, we observed in HEK293 cells expressing Smac MTS -hsCCS1-HA a transition from a slow-migrating band at ca . 60 kDa to a fast-migrating species at ca. 35 kDa via an intermediate band at 45 kDa ( Fig. 2g ). This result is consistent with the three expected forms of Smac MTS -hsCCS1-HA: a reduced immature form of Smac MTS -hsCCS1-HA, which still contains the unprocessed IMS-targeting signal (before import to the IMS, Fig. 2g ); a reduced form after the IMS-targeting signal has been cleaved (after import to IMS, Fig. 2g ); and an oxidized form ( Fig. 2e ). Processing of the IMS-targeting signal was completed within 20 min ( Supplementary Fig. S2 ), whereas reaching the oxidized form took between 1 and 2 h ( Fig. 2g ). In contrast, when we performed the experiment with hsCCS1-HA without the IMS-targeting signal, we did not observe any transition to a faster migrating form within the 2-h chase in our oxidation assay ( Fig. 2g ), that is, hsCCS1-HA did not become oxidized in the cytosol during this time. Taken together, we find that hsCCS1 becomes oxidized in the IMS within 2 h. In the cytosol, the protein becomes oxidized very inefficiently ( Fig. 2g ). The IMS localization of human CCS1 depends on cysteine 227 The difference between the hsCCS1 redox states in the cytosol and the IMS prompted us to investigate the importance of cysteine residues in the targeting of hsCCS1 to the IMS. We constructed six HEK293 cell lines expressing single or double cysteine mutants of hsCCS1-HA, which cover all nine cysteines of the protein (C12S, C22S/C25S, C113S, C141S/C144S, C227S and C244S/C246S). In whole-cell extracts, we did not observe significant differences in the expression levels of these proteins ( Fig. 3a ). Conversely, the level of hsCCS1(C227S)-HA was strongly decreased in the mitochondrial fraction ( Fig. 3b , down to about 27% of WT levels), whereas the levels of other cysteine mutants were either unchanged or slightly higher compared with levels observed in WT hsCCS1. This indicates that C227 is critical for the mitochondrial accumulation of hsCCS1. Importantly, C227 is not required for SOD1 activation, as a C227S mutant of CCS1 can still activate SOD1 in a S. cerevisiae model ( Supplementary Fig. S3 ). 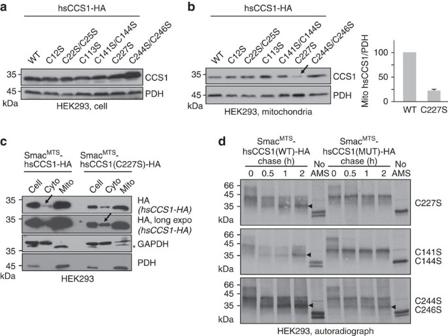Figure 3: Cysteine 227 is involved in mitochondrial accumulation of CCS1. (a) HEK293 cells that express different cysteine to serine mutants of hsCCS1-HA were analysed for the expression of hsCCS1-HA by western blotting. (b) Mitochondria were isolated from the cell lines introduced ina. Levels of hsCCS1-HA were analysed by western blotting. Mitochondrial levels of hsCCS1 and the C227S mutant were quantified and normalized by PDH amounts.n=2, error bars represent s.d. (c) Cytosolic and mitochondrial fractions were prepared from HEK293 cells producing SmacMTS-hsCCS1(C227S)-HA by differential centrifugation. Western blot analysis was performed using the indicated antibodies. Glyceraldehyde 3-phosphate dehydrogenase (GAPDH) and PDH served as cytosolic and mitochondrial loading controls, respectively. (d) HEK293 cells producing either SmacMTS-hsCCS1-HA or the C227S, C141S/C144S and C244S/C246S mutants were subjected to the oxidation assay as described inFig. 2. Original immunoblot images are shown inSupplementary Figs S7 and S8. Figure 3: Cysteine 227 is involved in mitochondrial accumulation of CCS1. ( a ) HEK293 cells that express different cysteine to serine mutants of hsCCS1-HA were analysed for the expression of hsCCS1-HA by western blotting. ( b ) Mitochondria were isolated from the cell lines introduced in a . Levels of hsCCS1-HA were analysed by western blotting. Mitochondrial levels of hsCCS1 and the C227S mutant were quantified and normalized by PDH amounts. n =2, error bars represent s.d. ( c ) Cytosolic and mitochondrial fractions were prepared from HEK293 cells producing Smac MTS -hsCCS1(C227S)-HA by differential centrifugation. Western blot analysis was performed using the indicated antibodies. Glyceraldehyde 3-phosphate dehydrogenase (GAPDH) and PDH served as cytosolic and mitochondrial loading controls, respectively. ( d ) HEK293 cells producing either Smac MTS -hsCCS1-HA or the C227S, C141S/C144S and C244S/C246S mutants were subjected to the oxidation assay as described in Fig. 2 . Original immunoblot images are shown in Supplementary Figs S7 and S8 . Full size image To characterize hsCCS1(C227S) further, we constructed a HEK293 cell line expressing Smac MTS -hsCCS1(C227S)-HA. Although the mitochondrial targeting of WT hsCCS1 with the Smac presequence was efficient ( Fig. 2a,b ), nearly half of the Smac MTS -hsCCS1(C227S)-HA localized to the cytosol ( Fig. 3c ). Moreover, Smac MTS -hsCCS1(C227S)-HA did not become oxidized during the 2-h chase in our oxidation assay ( Fig. 3d ), whereas the C244S/C246S mutant that we used as a control became similar to the oxidized WT. In addition, conversely to WT hsCCS1, Smac MTS -hsCCS1(C227S)-HA was not more oxidized than the respective MTS-less CCS1 variant ( Supplementary Fig. S4 ). We also observed that the IMS-targeting signal of Smac MTS -hsCCS1(C227S)-HA became completely processed within 20 min ( Fig. 3d and Supplementary Fig. S2 ), indicating that all Smac MTS -hsCCS1(C227S)-HA molecules, including those localized to cytosol, were initially imported to the IMS but could not be retained in this compartment. Notably, in the CCS1 crystal structure C227 forms a disulphide bond with C141 (ref. 23 ). When we tested the C141S/C144S mutant of Smac MTS -CCS1-HA, we found that it also did not become oxidized, indicating that in intact cells the C227–C141 disulphide is formed. Taken together, our data show that C227 and C141 (or C144) are important for disulphide bond formation of IMS-localized hsCCS1. Moreover, C227 is critical to accumulate and retain hsCCS1 in the IMS. IMS-targeted CCS1 drives IMS import of endogenous human CCS1 Which factors mediate C227-dependent IMS accumulation of hsCCS1? Mia40 is a primary candidate, because previously Kawamata and Manfredi [19] reported that transient cotransfection of Mia40 and CCS1 in COS cells increased the mitochondrial accumulation of this overproduced CCS1. We created HEK293 cells that stably express both Mia40-Strep and hsCCS1-HA. In this cell line, the expression of Mia40-Strep can be induced by doxycycline, while hsCCS1-HA is constitutively expressed. When, we compared the mitochondrial accumulation of hsCCS1-HA with or without the overexpression of Mia40, we were not able to observe significant differences ( Fig. 4a ). Thus, our results imply that in HEK293 cells, Mia40 overexpression has little effect on the distribution of hsCCS1. In addition, the absence of hsCCS1 import to mitochondria in S. cerevisiae ( Fig. 1d ) supports the notion that Mia40 is not likely the main factor for C227-dependent accumulation of hsCCS1. 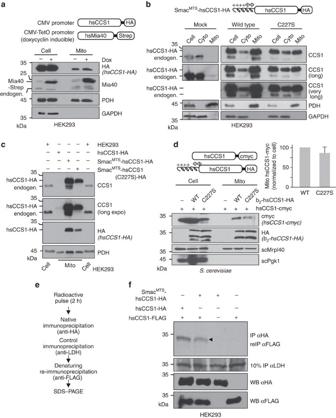Figure 4: IMS-localized hsCCS1 facilitates hsCCS1 import. (a) Mitochondria were isolated from HEK293 cells that constitutively produce hsCCS1-HA and express Mia40-Strep in a doxycycline-inducible manner. Expression of Mia40-Strep was induced by 1 μg ml−1doxycycline (Dox) for 24 h. Protein levels were analysed by western blotting. PDH and glyceraldehyde 3-phosphate dehydrogenase (GAPDH) served as loading controls. (b) Cytosolic and mitochondrial fractions were prepared by differential centrifugation from HEK293 cells expressing the empty vector (Mock), SmacMTS-hsCCS1-HA or SmacMTS-hsCCS1(C227S)-HA. Protein levels were analysed by western blotting against CCS1 (detection of endogenous CCS1 and CCS1-HA). PDH and GAPDH served as loading controls. (c) Mitochondria were isolated from HEK293 cell producing hsCCS1-HA, SmacMTS-hsCCS1-HA or SmacMTS-hsCCS1(C227S)-HA. Protein levels were analysed by western blotting against CCS1 (detection of CCS1 and CCS1-HA) and the HA tag (detection of CCS1-HA). PDH served as a loading control. Whole-cell extract of parental HEK293 was loaded next to those samples to indicate the size of endogenous hsCCS1. (d) hsCCS1-cmyc was coexpressed with either b2-hsCCS1-HA, b2-hsCCS1(C227S)-HA or an empty plasmid in cells of a Δccs1strain ofS. cerevisiae. Mitochondria were isolated from those strains and the levels of hsCCS1-cmyc were compared by western blotting. The mitochondrial cmyc signals were quantified and normalized to the cytosolic signals.n=2, error bars represent s.d. (e) Outline of the experimental procedure to detect interactions between mature and newly synthesized hsCCS1. HEK293 cells producing hsCCS1-HA or SmacMTS-CCS1-HA in combination with hsCCS1-FLAG were labelled with [35S] methionine for 2 h followed by chase periods with cold methionine of 0 or 2 h. Cells were lysed and protein complexes were isolated by native IP assay against the HA tag. Potentially coprecipitating hsCCS1-FLAG was subsequently isolated by denaturing IP assay against FLAG. Precipitates were analysed by SDS–PAGE and autoradiography. (f) Analysis of interaction between hsCCS1-HA and SmacMTS-CCS1-HA with hsCCS1-FLAG. The experiment was performed as described ine. Original immunoblot images are shown inSupplementary Figs S9 and S10. Figure 4: IMS-localized hsCCS1 facilitates hsCCS1 import. ( a ) Mitochondria were isolated from HEK293 cells that constitutively produce hsCCS1-HA and express Mia40-Strep in a doxycycline-inducible manner. Expression of Mia40-Strep was induced by 1 μg ml −1 doxycycline (Dox) for 24 h. Protein levels were analysed by western blotting. PDH and glyceraldehyde 3-phosphate dehydrogenase (GAPDH) served as loading controls. ( b ) Cytosolic and mitochondrial fractions were prepared by differential centrifugation from HEK293 cells expressing the empty vector (Mock), Smac MTS -hsCCS1-HA or Smac MTS -hsCCS1(C227S)-HA. Protein levels were analysed by western blotting against CCS1 (detection of endogenous CCS1 and CCS1-HA). PDH and GAPDH served as loading controls. ( c ) Mitochondria were isolated from HEK293 cell producing hsCCS1-HA, Smac MTS -hsCCS1-HA or Smac MTS -hsCCS1(C227S)-HA. Protein levels were analysed by western blotting against CCS1 (detection of CCS1 and CCS1-HA) and the HA tag (detection of CCS1-HA). PDH served as a loading control. Whole-cell extract of parental HEK293 was loaded next to those samples to indicate the size of endogenous hsCCS1. ( d ) hsCCS1-cmyc was coexpressed with either b 2 -hsCCS1-HA, b 2 -hsCCS1(C227S)-HA or an empty plasmid in cells of a Δ ccs1 strain of S. cerevisiae . Mitochondria were isolated from those strains and the levels of hsCCS1-cmyc were compared by western blotting. The mitochondrial cmyc signals were quantified and normalized to the cytosolic signals. n =2, error bars represent s.d. ( e ) Outline of the experimental procedure to detect interactions between mature and newly synthesized hsCCS1. HEK293 cells producing hsCCS1-HA or Smac MTS -CCS1-HA in combination with hsCCS1-FLAG were labelled with [ 35 S] methionine for 2 h followed by chase periods with cold methionine of 0 or 2 h. Cells were lysed and protein complexes were isolated by native IP assay against the HA tag. Potentially coprecipitating hsCCS1-FLAG was subsequently isolated by denaturing IP assay against FLAG. Precipitates were analysed by SDS–PAGE and autoradiography. ( f ) Analysis of interaction between hsCCS1-HA and Smac MTS -CCS1-HA with hsCCS1-FLAG. The experiment was performed as described in e . Original immunoblot images are shown in Supplementary Figs S9 and S10 . Full size image Another candidate for facilitating hsCCS1 import could be hsCCS1 molecules that are already present in their mature form inside the IMS. During SOD1 activation hsCCS1 forms heterodimers with SOD1 via its domain II, which is structurally homologous to SOD1 (refs 24 , 25 , 26 ; Fig. 1a ). It has been suggested that this mechanism not only mediates SOD1 folding in the cytosol but also drives SOD1 import into the IMS (refs 13 , 14 ). Moreover, during this activation by hsCCS1 a disulphide bond is introduced into SOD1. This disulphide bond encompasses the cysteine residues C146 and C57 in SOD1 that interestingly can be aligned with C227 and C141 in domain II of hsCCS1. In the hsCCS1 domain II crystal structure, these cysteines also form a disulphide bond [27] . As hsCCS1 can also form homodimers and a disulphide bond might have a role in mitochondrial accumulation of the protein, we speculated that IMS-localized hsCCS1 mediates the C227-dependent IMS accumulation of hsCCS1. To test this hypothesis, we assessed the localization of endogenous hsCCS1 in HEK293 expressing either Smac MTS -CCS1-HA or Smac MTS -CCS1(C227S)-HA. Strikingly, the accumulation of endogenous CCS1 in the mitochondria increased in HEK293 cells that expressed Smac MTS -CCS1-HA compared with the Mock situation and to cells expressing hsCCS1-HA ( Fig. 4b,c ). It is important to note that western blotting against HA detected only a single band for hsCCS1 compared with blotting with anti-CCS1, indicating that the lower band detected with anti-CCS1 indeed represents endogenous hsCCS1 ( Fig. 4c ). The accumulation of endogenous hsCCS1 depended on the presence of C227, because cells expressing Smac MTS -hsCCS1(C227S)-HA contain less endogenous hsCCS1 in the mitochondrial fraction compared with Smac MTS -hsCCS1-HA. However, in these cells endogenous hsCCS1 was enriched compared with the Mock situation, indicating that Smac MTS -hsCCS1(C227S), in principle, can facilitate hsCCS1 accumulation. The decreased enrichment compared with that of Smac MTS -hsCCS1-HA might thus, at least in part, also result from a failure of Smac MTS -hsCCS1(C227S)-HA to become retained in the mitochondria ( Fig. 3c ). As hsCCS1 is not imported into the S. cerevisiae mitochondria on its own, yeast cells represent an optimal system to further confirm that hsCCS1 becomes imported by already IMS-localized hsCCS1. Thus, we created a S. cerevisiae strain that coexpressed hsCCS1 and IMS-targeted hsCCS1. hsCCS1 was targeted specifically to the IMS by fusing it with the N-terminal 86 amino acids of cytochrome b 2 . To distinguish hsCCS1 with and without the targeting signal, these proteins were C-terminally tagged with an HA ( b 2 -hsCCS1-HA) and a cmyc tag (hsCCS1-cmyc), respectively. As expected, when hsCCS1-cmyc was expressed alone, we were not able to detect any hsCCS1-cmyc in mitochondrial fractions ( Fig. 4d ). In contrast, when b 2 -hsCCS1-HA was coexpressed, hsCCS1-cmyc was detected in the mitochondrial fraction. We observed less mitochondrial hsCCS1-cmyc with b 2 -hsCCS1(C227S)-HA ( Fig. 4d ), and none at all when we coexpressed hsCCS1-cmyc with IMS-targeted scCCS1 ( b 2 -scCCS1) ( Supplementary Fig. S5 ). It is important to note that in contrast to mammalian cells, in our heterologous yeast system the IMS-targeted C227S can efficiently facilitate hsCCS1 accumulation in the IMS (compare Fig. 4b,d ). This could, for example, stem from differences in the system (yeast versus mammalian cells) and/or the fact that we compare the accumulation of endogenous human CCS1 (human cells) with the accumulation of overexpressed human CCS1 (yeast cells). If import of hsCCS1 into the IMS depends on hsCCS1 that is already present in the IMS, we would expect that newly synthesized hsCCS1 transiently interacts with mitochondrial hsCCS1. To investigate such an interaction, we constructed HEK293 cell lines that coexpressed hsCCS1-FLAG with either hsCCS1-HA or with Smac MTS -hsCCS1-HA. We then employed a pulse-chase assay followed by an immunoprecipitation (IP)/re-IP approach ( Fig. 4e ). In this assay, newly synthesized proteins, including hsCCS1-FLAG, are first radioactively labelled. Subsequently, a native IP assay against HA is performed, which leaves potential complexes between (Smac MTS -)hsCCS1-HA and hsCCS1-FLAG intact. Then, the precipitated lysate is analysed by a denaturing re-IP assay against FLAG. To prove the equal use of cells, an IP assay against lactate dehydrogenase is performed. We thereby found that newly synthesized hsCCS1-FLAG interacted with both hsCCS1-HA and Smac MTS -hsCCS1-HA ( Fig. 4f ). Taken together, our data indicate that the import of hsCCS1 into the IMS depends on the interaction with hsCCS1 molecules that already are in the IMS. On the basis of our results, we propose a novel pathway for protein import into the IMS of human cells. Thereby, IMS-localized hsCCS1 serves as an import receptor for the import of immature hsCCS1 ( Fig. 5a ). We propose that hsCCS1 is imported from the cytosol into the IMS in its unfolded and reduced form. Domain II of IMS-localized hsCCS1 interacts with incoming unfolded hsCCS1, and as a result hsCCS1 becomes folded and oxidized. Our model is supported by the fact that the overexpression of IMS-targeted WT hsCCS1 increased the IMS localization of endogenous hsCCS1 ( Fig. 4b,c ), and that in yeast the sole expression of IMS-targeted hsCCS1 resulted in a mitochondrial accumulation of hsCCS1 ( Fig. 4d ). Moreover, we demonstrated an interaction between newly synthesized hsCCS1 and mature hsCCS1 ( Fig. 4f ). Importantly, we found this interaction between cytosolic hsCCS1 variants as well, suggesting that the interaction with mature hsCCS1 might be a general feature of hsCCS1 maturation in the cytosol and in the IMS. We propose that only hsCCS1 molecules that in the cytosol avoid the initial interaction with mature hsCCS1 remain competent for import into the IMS. 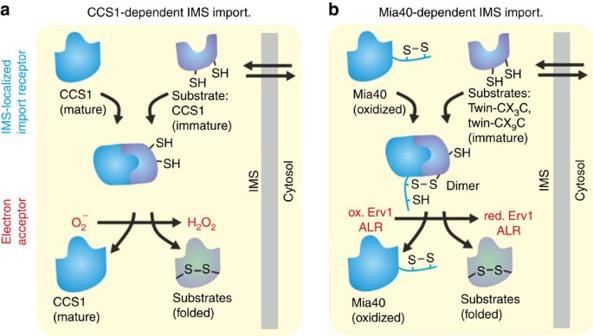Figure 5: A novel pathway for protein import into the mitochondrial intermembrane space. (a) Mitochondrial import by hsCCS1. Unfolded and reduced hsCCS1 interacts with IMS-localized mature hsCCS1 via its domain II. Immature hsCCS1 becomes oxidized and folded in the course of this interaction and thereby trapped in the IMS. ROS likely contribute the oxidative power for this process. A role of Mia40 in hsCCS1 import cannot be formally excluded, although Mia40 overexpression does not influence mitochondrial hsCCS1 levels. (b) Mitochondrial import by the oxidoreductase Mia40 and the sulphydryl oxidase Erv1/ALR. Unfolded and reduced precursors interact with Mia40 and thereby become oxidized and folded. The oxidative power derives from interaction of Mia40 with the mitochondrial sulphydryl oxidase Erv1/ALR. Figure 5: A novel pathway for protein import into the mitochondrial intermembrane space. ( a ) Mitochondrial import by hsCCS1. Unfolded and reduced hsCCS1 interacts with IMS-localized mature hsCCS1 via its domain II. Immature hsCCS1 becomes oxidized and folded in the course of this interaction and thereby trapped in the IMS. ROS likely contribute the oxidative power for this process. A role of Mia40 in hsCCS1 import cannot be formally excluded, although Mia40 overexpression does not influence mitochondrial hsCCS1 levels. ( b ) Mitochondrial import by the oxidoreductase Mia40 and the sulphydryl oxidase Erv1/ALR. Unfolded and reduced precursors interact with Mia40 and thereby become oxidized and folded. The oxidative power derives from interaction of Mia40 with the mitochondrial sulphydryl oxidase Erv1/ALR. Full size image The importance of domain II of hsCCS1 is emphasized by the fact that a cysteine mutation in this domain (C227) affected the localization of hsCCS1. Although our data do not exclude the possibility that C227 is involved in an intermolecular interaction with another hsCCS1 molecule, we propose that C227 facilitates the folding of newly imported hsCCS1 by forming an intramolecular disulphide bond, thereby preventing a backsliding to the cytosol (folding trap model). The proposed role of C227 in mitochondrial import is supported by the following results. First, hsCCS1(C227S) does not efficiently accumulate in the mitochondria ( Fig. 3b ). Second, significant amounts of hsCCS1(C227S) accumulate in the cytosol, even if it had been targeted to the mitochondria ( Fig. 3c ). Third, in the crystal structure of hsCCS1, C227 forms a disulphide bond with C141 (ref. 23 ). Fourth, hsCCS1 is oxidized in the IMS ( Fig. 2d,e,g ). Finally, Smac MTS -hsCCS1 but not Smac MTS -hsCCS1(C227S) or Smac MTS -hsCCS1(C141S/C144S) become oxidized after synthesis ( Fig. 3d ). These findings also indicate that C227 forms a disulphide bond with either C141 or C144. This is supported by the crystal structure in which C227 forms a disulphide bond with C141 (ref. 23 ). Interestingly, mutation of C141/C144 however does not impair IMS import of hsCCS1. It might thus be possible that C227 is mainly important to mediate an initial interaction with preexisting hsCCS1 so as to allow time for folding of domain II and retention in the IMS. In the WT a disulphide bond is subsequently formed, whereas in the C141S/C144S double mutant folded hsCCS1 is released and remains in the IMS in a reduced state. The import system for hsCCS1 resembles the import pathway for small cysteine-containing proteins by the mitochondrial disulphide relay/Mia40 system [18] , [28] ( Fig. 5 ). Both systems rely on import receptors in the IMS (CCS1 and Mia40, respectively). These receptors serve as chaperones that mediate protein folding and thereby trap substrate proteins in the IMS. Importantly, although import by both pathways usually relies on concomitant disulphide bond formation, the machineries are also capable of importing certain proteins in a cysteine-independent manner. For Mia40, this has recently been demonstrated for a cysteine-free variant of the substrate Atp23 (ref. 29 ). In the case of the CCS1-dependent pathway, WT scCCS1 and scCCS1(C27S/C64S) constitute such substrates. Both proteins accumulate in human mitochondria, although they do not contain the cysteine corresponding to the position of C227. In some species, including Arabidopsis, Sc. pombe and N. crassa , CCS1 lacks both, equivalents for the cysteines 27 and 64 in domain I and for C227 in domain II ( Fig. 1b ). We speculate that in these species, CCS1s are imported by domain II interactions as well. Many proteins of the recently identified yeast IMS proteome [30] neither contain presequences nor clear Mia40 recognition motifs. Some of these substrates and their human homologues might also be imported by a folding trap mechanism but in a Mia40-independent manner, some might even be by the action of hsCCS1. The oxidation of hsCCS1 in the IMS requires an electron acceptor. Kawamata and Manfredi [19] reported that treatment of cells by the complex III inhibitor, antimycin A resulted in an increased IMS accumulation of CCS1. Antimycin A treatment is known to increase superoxide production at complex III, especially towards the IMS [1] . We confirmed these findings in HEK293 cells, and in addition found that antimycin A-dependent accumulation was limited to hsCCS1-HA and did not occur for the C227S mutant, again highlighting the importance of this residue for mitochondrial accumulation ( Supplementary Fig. S6 ). This might indicate that oxidative stress has a role in the formation of the disulphide bonds in hsCCS1 and thereby influences the IMS localization of hsCCS1 and therefore SOD1 activity. Human cell lines Flp-In T-Rex-293 (FT293) cells were obtained from Invitrogen and were cultured in DMEM (PAA) supplemented with 10% fetal bovine serum (PAA), penicillin and streptomycin (PAA), and 15 μg ml −1 blasticidin (InvivoGen, San Diego, CA). For stably transfected FT293 cells, 50 μg ml −1 hygromycin B (PAA) was added. Doxycycline was obtained from Sigma. To construct stable cell lines, FT293 cells were transfected with 900 ng pOG44 plasmid (Invitrogen) and 100 ng pcDNA5-derived plasmids. For primers and plasmids, see Supplementary Table S1 . Cells were selected in media containing 50 μg ml −1 hygromycin B. Protein production was induced by the addition of 1 μg ml −1 doxycycline. For the stable cell line expressing both Mia40-strep and hsCCS1-HA, FT293 cells were first transfected with pcDNA5-Mia40-strep and selected by hygromycin B. The resulting cell line was transfected with pcDNA3-hsCCS1-HA and selected using 400 μg ml −1 Geneticin (Invitrogen). Yeast strains The Δccs1 strain was derived from the WT strain YPH499 ( MATa ura3-52 lys2-801_amber ade2-101_ochre trp1-Δ63 his3-Δ200 leu2-Δ1 ) by a replacement of the CCS1 open reading frame with a URA3 cassette 3. The Δccs1 strains expressing CCS1 variants were generated by transformation with the respective plasmids. Strains were grown in S(Lac) medium (0.85% yeast nitrogen base, 2.5% (NH 4 ) 2 SO 4 , 9.9% lactate, 20 mg l −1 adenine sulphate, 20 mg l −1 uracil, 100 mg l −1 L -leucine, 30 mg l −1 L -lysine and 20 mg l −1 L -histidine, pH 5.5) with 0.2% galactose at 30 °C. Cloning and antibodies For primers and plasmids, see Supplementary Table S1 . The following antibodies were used: anti-MrpL40 (1:1,000) [7] , anti-Pgk1 (Invitrogen, 459,250, 1:10,000), anti-scCCS1 (1:1,000) [7] , anti-hsCCS1 (Santa Cruz, sc-58340 1:200; Abcam, ab16964, 1:2,000), anti-glyceraldehyde 3-phosphate dehydrogenase (Abcam, ab8245, 1:500), anti-lactate dehydrogenase (Santa Cruz, sc-133123, 1:100), anti-PDH (Santa Cruz, sc-65242, 1:200), anti-Smac/Diablo (Prosci, 2,411, 1:1,000), anti-HA (Sigma, H3663, 1:1,000) and anti-cMyc (Santa Cruz, sc-40, 1:200). The antibody directed against human Mia40 was raised in rabbits injected with the purified full-length protein (1:1,000). Subcellular fractionation and isolation of mitochondria Mitochondrial isolation from HEK293 cells was performed as described [31] . In short, cells were homogenized on ice with a Potter–Elvehjem homogenizer in a buffer consisting of 2 mM KCl, 1.5 mM MgCl, 1 mg ml −1 BSA and 20 mM HEPES, pH 8.0. The homogenate was centrifuged at 1,600 g for 10 min at 4 °C. The pellet consisting of nuclei and unbroken cells was discarded, and the supernatant was centrifuged at 9,000 g for 15 min at 4 °C, and washed four times with buffer consisting of 210 mM mannitol, 70 mM sucrose, 2 mM EDTA, 500 mM KCl and 20 mM HEPES, pH 8.0. The pellet was resuspended in the same buffer with KCl omitted and was immediately incubated at room temperature for 15 min with 100 μg ml −1 proteinase K. Protease digestion was stopped by the addition of 3 mM phenylmethyl sulphonyl fluoride, and incubation was continued for 5 min at room temperature. For subcellular fractionation of HEK293 cells by digitonin titration, cells were treated with ice-cold fractionation buffer (20 mM HEPES, pH 7.4, 250 mM sucrose, 50 mM KCl, 2.5 mM MgCl, 1 mM dithiothreitol) containing 0.005, 0.03, 0.3 or 0% digitonin for 30 min at 4 °C. Samples were centrifuged at 1,000 g for 5 min and supernatants were analysed by SDS–PAGE. Isolation of the mitochondria from S. cerevisiae was performed as described [7] . In short, after cell walls were broken by Zymolyase treatment, cells were homogenized on ice with a Potter–Elvehjem homogenizer in a buffer consisting of 0.6 M sorbitol, 1 mM EDTA and 10 mM Tris-HCl (pH 7.4). The homogenate was centrifuged at 2,000 g for 5 min at 4 °C. The pellet consisting of nuclei and unbroken cells was discarded, and the supernatant was centrifuged at 17,000 g for 12 min at 4 °C, and washed four times with buffer consisting of 0.6 M sorbitol and 20 mM HEPES, pH 8.0. The pellet was resuspended in the same buffer and was immediately incubated at room temperature for 15 min with 100 μg ml −1 proteinase K. Protease digestion was stopped by the addition of 3 mM phenylmethyl sulphonyl fluoride, and incubation was continued for 5 min at room temperature. In vivo redox state analyses To determine the redox state of CCS1 in HEK293 cells, cells were grown to ~ 80% confluency. The medium was removed, cells were treated with 10% trichloroacetic acid (TCA), and were scratched off and pelleted by centrifugation. The TCA pellet was resuspended in 40 μl AMS buffer (58 mM Tris, pH 7.0, 7% glycerol, 1.5% SDS, 0.1% bromcresol purple) containing 15 mM AMS in case of AMS modification. Modification took place for 1 h at 25 °C in the dark. Pulse-chase oxidation assay Cells were starved with cysteine and methionine-free medium (Sigma) for 15 min at 37 °C and were pulse-labelled for 5 min at 37 °C with medium containing [ 35 S]-methionine at a concentration of 200 μCi ml −1 (Perkin Elmer). Pulse labelling was stopped by adding the chase medium containing 20 mM methionine. After variable times at 37 °C, the chase was stopped by adding ice-cold 8% TCA. TCA precipitation was performed by centrifugation at 13,000 g for 15 min and washing with 5% ice-cold TCA. Protein precipitates were dissolved in 0.2 M Tris, pH 7.5, 6 M urea, 10 mM EDTA and 2% SDS. Samples were modified with 15 mM AMS for 1 h at 20 °C. After modification, samples were filled to 250 μl using buffer A (30 mM TrisCl, pH 8, 100 mM NaCl, 5 mM EDTA and 2% SDS) and were incubated for 5 min at 96 °C. Then, 750 μl of buffer B (buffer A without SDS and containing 2.5% Triton X-100) was added and the mixture was incubated at 4 °C for 1 h. Samples were cleared by centrifugation at 25,000 g for 1 h. The supernatant was subjected to IP assay with antibodies conjugated to protein A beads at 4 °C over night. Samples were washed four times using buffer C (buffer A without SDS and containing 1% Triton X-100) and once using buffer D (30 mM TrisCl, pH 8, 100 mM NaCl and 5 mM EDTA). Proteins were eluted by adding Laemmli buffer (2% SDS, 60 mM Tris, pH 6.8, 10% glycerol and 0.0025% bromophenol blue) to the dried beads and subsequent boiling for 5 min at 95 °C. Samples were analysed by SDS–PAGE and autoradiography. How to cite this article: Suzuki, Y. et al. Human copper chaperone for superoxide dismutase 1 mediates its own oxidation-dependent import into mitochondria. Nat. Commun. 4:2430 doi: 10.1038/ncomms3430 (2013).